Familial Alzheimer’s mutations within APPTM increase Aβ42 production by enhancing accessibility of ε-cleavage site The high Aβ42/Aβ40 production ratio is a hallmark of familial Alzheimer’s disease, which can be caused by mutations in the amyloid precursor protein (APP). The C-terminus of Aβ is generated by γ-secretase cleavage within the transmembrane domain of APP (APPTM), a process that is primed by an initial ε -cleavage at either T48 or L49, resulting in subsequent production of Aβ42 or Aβ40, respectively. Here we solve the dimer structures of wild-type APPTM (AAPTM WT) and mutant APPTM (FAD mutants V44M) with solution NMR. The right-handed APPTM helical dimer is mediated by GXXXA motif. From the NMR structural and dynamic data, we show that the V44M and V44A mutations can selectively expose the T48 site by weakening helical hydrogen bonds and increasing hydrogen–deuterium exchange rate ( k ex ). We propose a structural model in which FAD mutations (V44M and V44A) can open the T48 site γ -secretase for the initial ε -cleavage, and consequently shift cleavage preference towards Aβ42. Amyloid β-peptide (Aβ) is the major component of senile plaques, a pathologic hallmark of Alzheimer’s disease (AD) [1] . Amyloid precursor protein (APP) is an integral membrane protein with a single transmembrane (TM) domain, which is consecutively cleaved by β- and γ-secretase to generate amyloid beta (Aβ) peptides [2] . Aβ40 and Aβ42, consisting of 40 and 42 residues, respectively, are the two major isoforms of Aβ in human brains [1] , [3] . While Aβ40 is relatively benign, Aβ42 aggregates rapidly into neurotoxic oligomers and fibrils (plaques) [4] . Aβ42 is not only toxic in neuronal culture [5] , but also in animal models [6] . Familial Alzheimer’s disease (FAD) is caused by dominant mutations in genes encoding APP and γ-secretase. FAD is biochemically characterized by the increased ratio of Aβ42 over Aβ40 (refs 7 , 8 ), implicating the crucial role of Aβ42 in AD pathogenesis. However, the mechanism of how FAD mutations increase Aβ42/Aβ40 remains poorly understood. The proteolytic cleavage of APP is initiated by β-secretase within the extracellular domain of APP, releasing a C-terminal membrane-anchored fragment of 99 residues (C99) [9] , [10] . C99 is further processed by γ-secretase within the TM domain of APP (APPTM) to yield mature Aβ peptides and the APP intracellular domain (AICD) [11] , [12] , [13] . However, the cleavage of APPTM by γ-secretase is not specific, as varying lengths of Aβ peptides have been observed [11] . Aβ40 is the predominant product, while Aβ42 is generated to a lesser extent [4] . Another cleavage site, called the ε-cleavage site, has recently been established as the initial C99 cleavage site by γ-secretase, which generates Aβ48 or Aβ49 and AICD49-99 or AICD50-99, respectively [14] . Successive proteolysis by the processive carboxypeptidase-like activity of γ-secretase releases tripeptides and tetrapeptides from the C-terminus of Aβ48 and Aβ49. Two production lines are distinguished, one for Aβ40 and the other for Aβ42. Aβ46, Aβ43 and Aβ40 are generated from Aβ49, while Aβ45, Aβ42 and Aβ38 are produced from Aβ48 (ref. 14 ). Therefore, initial ε-cleavage at residue 48 (T48, γ-secretase cleaving between residues 48 and 49) or 49 (L49, cleaving between 49 and 50) determines whether Aβ42 or Aβ40, respectively, can be produced and can critically influence the Aβ42/40 ratio. Twelve FAD mutations have been identified within the APPTM [7] , [15] , [16] , [17] , [18] , [19] , [20] , which contains the ε- and γ-cleavage sites. These FAD mutations contribute to an increased Aβ42/Aβ40 ratio [8] , [21] . Using APPTM as the substrate, we have developed a novel γ-secretase assay which reproduces Aβ42/Aβ40 ratios for WT APPTM and FAD mutants [22] . This suggests that APPTM itself, as a substrate for γ-secretase, mimics the behaviour of the natural substrate C99 and that APPTM plays an important role in determining Aβ42/Aβ40 ratios. Although ample structural work on APPTM has been published, it remains unclear how FAD mutation within APPTM increase the Aβ42/Aβ40 ratio. Sanders’ group presented the first solution NMR studies of C99 (refs 23 , 24 ), which includes APPTM, and a recent monomer structure relevant for cholesterol binding [23] . However, the existence of APPTM as a dimer has been supported by numerous studies [24] , [25] , [26] , [27] , [28] . Sato et al . [27] derived a dimeric structural model for APPTM based on limited constraints from solid-state NMR. Solid-state NMR also revealed both helical and non-helical conformations at the two termini and in the vicinity of the γ-secretase site in APPTM in lipids [29] . Computational models of APPTM dimers were published by Miyashita et al . [30] and more recently by Wang et al . [31] Finally, Nadezhddin et al . [28] reported the solution NMR structure of APPTM WT as a left-handed dimer, though this model is based on intermolecular NOEs from filtered experiments only and has not been refined with residual dipolar couplings (RDCs). In this study, to explore the structural mechanism of increased Aβ42/Aβ40 ratio in FAD mutations within APPTM, we use solution NMR spectroscopy to investigate the structure and dynamics of three variants of APPTM, wild type (WT) and two FAD mutants, V44M (French mutation) and V44A (German mutation). Because we have shown APPTM itself is an excellent substrate of γ-secretase and FAD mutations within APPTM produce similar effects on 42/40 ratios as in assays using C99 as the substrate [22] , our NMR studies of APPTM itself can be directly correlated to the specificity of γ-secretase cleavage and Aβ42/Aβ40 ratios. Here, we show that V44M and V44A significantly alter the structure and dynamics of T48, the ε-cleavage site for Aβ42 production and propose a novel mechanism for increased Aβ42/Aβ40 ratio in FAD. V44M and V44A cause large CSP at the ε-cleavage site T48 Isotopically labelled APPTM WT V44M were reconstituted in dodecylphosphocholine (DPC) micelles as described in Chen et al . [32] and their complete assignments have been achieved with triple resonance experiments and deposited in BioMagResBank (BMRB entry 18,648 and 18,649). The residues are numbered according to Aβ ( Supplementary Fig. S1 ). 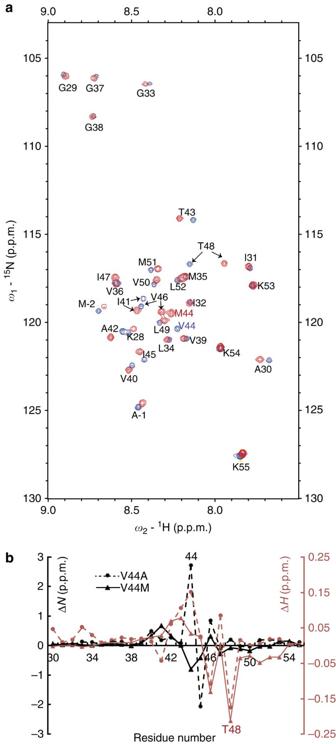Figure 1: FAD mutations within APPTM of V44M and V44A cause large changes in amide proton chemical shift of T48. (a)15N-H HSQC of APPTM WT (blue peaks), overlaid with that of V44M (red peaks). Residues M-2 and A-1 are non-APPTM residues N-terminal to APPTM due to cloning. (b) CSP caused by V44M (▲ joined by solid lines) and V44A (●joined by dashed lines) in amide proton (red) and nitrogen (black). Residues are numbered according to Aβ for easy correlation with Aβ production (Supplementary Fig. S1). In both FAD mutants, largest proton CSP occurs at T48. While the proton CSP pattern is similar to V44M, V44A causes larger nitrogen CSP at residues 44–46. Average backbone nitrogen chemical shifts of V, M, A are 121.08, 120.07 and 123.22 p.p.m., respectively, which mirrors the larger and opposite change in15N CSP at residue 44 in V44A compared with V44M. Figure 1a shows the 15 N– 1 H HSQC spectra of WT and V44M APPTM, with narrow dispersion typical of TM helices. The two spectra have similar peak patterns, suggesting that the V44M mutation does not change the overall fold of APPTM. Large chemical shift perturbations (CSPs) are observed at and near the site of the mutation (residues 44–48), as expected ( Fig. 1b ). While the largest 15 N CSP is at V44M, the largest 1 H CSP occurs at T48 ( Fig. 1b ), whose amide proton chemical shift decreases from 8.14 p.p.m. in WT to 7.93 p.p.m. in the mutant. The ~0.2 p.p.m. CSP indicates significant changes in magnetic environment of T48 amide proton, most likely due to changes in hydrogen bonding. We also have compared the backbone amide chemical shifts of V44A, another FAD mutant, with WT ( Fig. 1b ). While the largest 15 N CSP is at the site of mutation V44A, the largest 1 H CSP again occurs at T48 ( Fig. 1b ). As T48 is the initial recognition site of γ-secretase for the Aβ42 production line ( Supplementary Fig. S1 ) [14] , such changes in the local conformations of the ε-cleavage site may have important implications for the Aβ42/Aβ40 ratio. Figure 1: FAD mutations within APPTM of V44M and V44A cause large changes in amide proton chemical shift of T48. ( a ) 15 N-H HSQC of APPTM WT (blue peaks), overlaid with that of V44M (red peaks). Residues M-2 and A-1 are non-APPTM residues N-terminal to APPTM due to cloning. ( b ) CSP caused by V44M (▲ joined by solid lines) and V44A ( ● joined by dashed lines) in amide proton (red) and nitrogen (black). Residues are numbered according to Aβ for easy correlation with Aβ production ( Supplementary Fig. S1 ). In both FAD mutants, largest proton CSP occurs at T48. While the proton CSP pattern is similar to V44M, V44A causes larger nitrogen CSP at residues 44–46. Average backbone nitrogen chemical shifts of V, M, A are 121.08, 120.07 and 123.22 p.p.m., respectively, which mirrors the larger and opposite change in 15 N CSP at residue 44 in V44A compared with V44M. Full size image V44M changes local conformations of ε-cleavage sites To further investigate the detailed structural changes brought about by the V44M mutation, we solved the solution structures of both APPTM WT and V44M dimers, which were based on unambiguous intermolecular NOEs ( Fig. 2 ) and RDCs from two different alignment media ( Table 1 ). The dimerization of APPTM in DPC micelles was confirmed by analytical ultracentrifugation ( Supplementary Fig. S2 ) and supported by numerous previous studies [24] , [25] , [26] , [27] , [28] . Unambiguous intermolecular NOEs were determined by a number of chimera NMR samples with selective isotopical labelling ( Fig. 2 ). Because only one set of NMR resonances are observed ( Fig. 1a ), the structure was calculated as a symmetric dimer. On average, 25.4 (WT) and 25.9 (V44M) constraints per residue were obtained, including 9 intermolecular NOEs for WT and 11 intermolecular NOEs for V44M. An ensemble of 20 structures were calculated from XPLOR-NIH for WT and V44M (for stereo images of superimposed NMR structures, see Supplementary Figs S3 and S4 ), with backbone and heavy atom pairwise RMSDs at 0.79 and 1.28 Å (WT) and 0.81 and 1.31 Å (V44M), respectively ( Table 1 ). The coordinates and constraints have been deposited in the protein data bank as 2LZ3 (WT) and 2LZ4 (V44M). 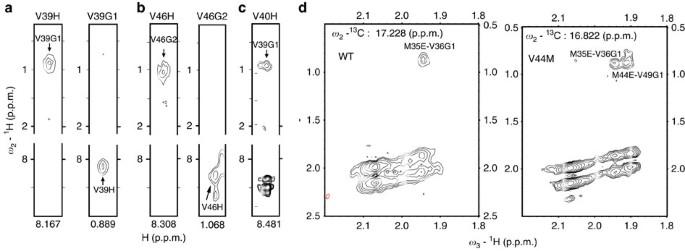Figure 2: Unambiguous determination of intermolecular NOEs. Reciprocal intermolecular NOE peaks between V39HN and V39HG1 (a), and between V46HN and V46HG2 (b), detected in a 1:1 mixed sample of uniformly13C labelled APPTM and uniformly15N labelled APPTM, yielding unambiguous intermolecular NOEs between13C-H and15N-H. The left panel is the strip from13C-selected15N-NOESY, while the right panel is the strip from15N-selected13C-NOESY. (c) V40HN-V39G1 intermolecular NOE detected in a 1:1 mixed sample of uniformly15N-labelled and perdeuterated V44M, and natural abundance V44M, by 3D15N-NOESY, giving rise to the intermolecular NOEs between15N-H and aliphatic protons. (d) Intermolecular NOEs detected by filtered13C-NOESY in a 1:1 mixed sample of13C,15N-APPTM and unlabelled APPTM. A new intermolecular NOEs M44E-V49G1 appears in the V44M mutant. Figure 2: Unambiguous determination of intermolecular NOEs. Reciprocal intermolecular NOE peaks between V39HN and V39HG1 ( a ), and between V46HN and V46HG2 ( b ), detected in a 1:1 mixed sample of uniformly 13 C labelled APPTM and uniformly 15 N labelled APPTM, yielding unambiguous intermolecular NOEs between 13 C-H and 15 N-H. The left panel is the strip from 13 C-selected 15 N-NOESY, while the right panel is the strip from 15 N-selected 13 C-NOESY. ( c ) V40HN-V39G1 intermolecular NOE detected in a 1:1 mixed sample of uniformly 15 N-labelled and perdeuterated V44M, and natural abundance V44M, by 3D 15 N-NOESY, giving rise to the intermolecular NOEs between 15 N-H and aliphatic protons. ( d ) Intermolecular NOEs detected by filtered 13 C-NOESY in a 1:1 mixed sample of 13 C, 15 N-APPTM and unlabelled APPTM. A new intermolecular NOEs M44E-V49G1 appears in the V44M mutant. Full size image Table 1 NMR and refinement statistics for APPTM structures. Full size table Both WT and V44M form right-handed dimers, as in the classical TM dimer of glycophorin A (GpA) ( Fig. 3 ) [33] . The crossing angle between the two helices is 22° for WT and 33° for V44M. For both APPTM WT and V44M, the GXXXA motif (residues 38–42) mediates the dimer interface ( Fig. 3a ). In contrast, the GXXXG motifs in APPTM do not have a direct role in dimerization. In addition, the side chains of M35, V39, I45, V46 and L49 provide key hydrophobic interactions at the dimer interface for the WT molecule. There is no hydrogen bond or salt bridge across the dimer interface. 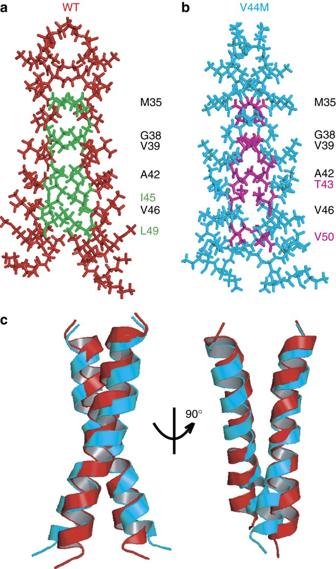Figure 3: NMR structures and dimer interfaces of WT and V44M. The interface residues are colored green in WT structure (a) and magneta in V44M structure (b). Interfacial residues unique to WT is labelled in green letters while those unique to V44M is labelled in magenta. GXXXA is the dimerization motif in both structures, but the interface is shifted towards the C-terminus in V44M. (c) Overlay of the ribbon representation of structures of WT (red) and V44M (blue). V44M conserves the overall dimer fold, with an RMSD between the average structures of WT and V44M of 2.4 Å. Figure 3: NMR structures and dimer interfaces of WT and V44M. The interface residues are colored green in WT structure ( a ) and magneta in V44M structure ( b ). Interfacial residues unique to WT is labelled in green letters while those unique to V44M is labelled in magenta. GXXXA is the dimerization motif in both structures, but the interface is shifted towards the C-terminus in V44M. ( c ) Overlay of the ribbon representation of structures of WT (red) and V44M (blue). V44M conserves the overall dimer fold, with an RMSD between the average structures of WT and V44M of 2.4 Å. Full size image The dimer fold and interface are generally retained in the V44M mutant but the dimerization pattern is altered significantly ( Fig. 3b ). The GXXXA motif and the side chains of M35, V39 and V46 still mediate dimerization; however, there is a registry shift in hydrophobic side-chain packing towards the C-terminus. I45 and L49 are no longer present at the dimer interface in V44M while T43 and V50 provide new hydrophobic packing for V44M dimerization. While T48 is not at the dimer interface in either structure, V44M mutation relocates L49 away from the dimer interface. The large CSP in the T48 amide proton led us to more closely examine the helical hydrogen bonds. Overall, the V44M mutation strengthens hydrogen bonding at the N-terminal half of the helix while weakening those at the C-terminal half ( Fig. 4 ). The helical hydrogen bonds involving the ε-cleavage site T48 and L49 amides experience large changes. In the 20 NMR structures, the average distance between the T48 amide proton and the V44 carbonyl oxygen is 2.2±0.2 Å and 3.23±0.14 Å in the WT and V44M mutant, respectively. The average distance between the L49 amide proton and the I45 carbonyl oxygen is 2.3±0.2 Å and 2.8±0.4 Å in WT and V44M, respectively. Thus the helical hydrogen bond involving both T48 and L49 amide protons are both weakened and the effect is much more pronounced for T48 than for L49. 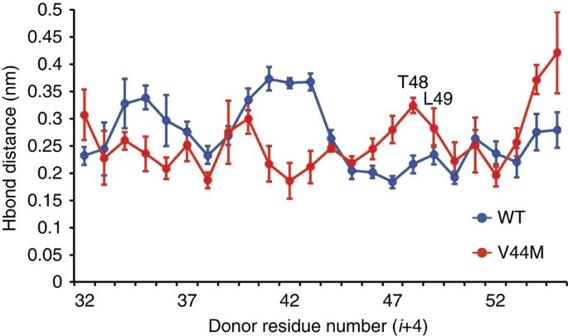Figure 4: Average length of helical hydrogen bonds in APPTM WT and V44M. The average distances between the donor amide proton (residuei+4) and the acceptor carbonyl (residuei) in the TM helix in the 20 NMR structures and their standard deviations are plotted versus residue number of the donor amide. The error bars here are standard deviations of hydrogen bond lengths derived from 20 NMR structures. Overall, hydrogen bonds at the N-terminal half become shorter while hydrogen bonds at the C-terminal half become longer in V44M, suggesting that the V44M mutation tightens up the N-terminal half helix while loosening up the C-terminal half helix. In particular, the helical hydrogen bond involving T48 amide is significantly lengthened, consistent with its decreased amide chemical shift in V44M. Figure 4: Average length of helical hydrogen bonds in APPTM WT and V44M. The average distances between the donor amide proton (residue i +4) and the acceptor carbonyl (residue i ) in the TM helix in the 20 NMR structures and their standard deviations are plotted versus residue number of the donor amide. The error bars here are standard deviations of hydrogen bond lengths derived from 20 NMR structures. Overall, hydrogen bonds at the N-terminal half become shorter while hydrogen bonds at the C-terminal half become longer in V44M, suggesting that the V44M mutation tightens up the N-terminal half helix while loosening up the C-terminal half helix. In particular, the helical hydrogen bond involving T48 amide is significantly lengthened, consistent with its decreased amide chemical shift in V44M. Full size image V44M and V44A enhance k ex of T48 more than L49 To further probe helical stability and dynamics with residue-specific resolution, we have carried out hydrogen–deuterium (HD) exchange measurements at 298 K ( Fig. 5a ). Helical core residues between I41 and I47 had no decrease in their signal intensity in HSQC spectra after 30 h in D 2 O, due to very slow exchange with water, in both WT and V44M ( Fig. 5a and Supplementary Fig. S5 ). Residues V36–V40 display decreasing exchange rates towards the centre of the helix while exchange rates of residues T48–V50 increase towards the C-terminus in both WT and V44M. T48 has an ~4-fold enhancement in HD exchange rate, increasing from 0.009 per h in WT to 0.034 per h in V44M ( Figs 4 and 5a ), while L49 has an ~2-fold increase (0.028 per h in WT versus 0.05 per h in V44M) ( Fig. 5a ). Consequently, both initial ε-cleavage sites are destabilized by V44M, but the effect is more significant for T48 than for L49. Titration with paramagnetic relaxation enhancement (PRE) probes demonstrated similar micelle embedment around the ε-cleavage sites in WT and V44M ( Supplementary Fig. S6 ), suggesting the observed changes in HD exchange rates are not due to the differences in micelle embedment. 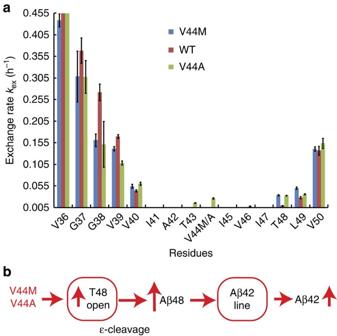Figure 5: HD exchange shows that FAD mutants V44M and V44A destabilize the local conformations of T48 more than L49. (a) HD exchange rates for slowly exchanging residues in WT APPTM, V44M and V44A are plotted. Terminal residues (K28-M35 and L52-K55) exchange with D2O completely within 1 h (kex>5 per h) and their rates are not plotted. Exchange rates for T48 are significantly enhanced by V44A and V44M mutations while the increases for L49 are to a lesser extent. Increasedkexvalues at A44 and T43 are likely due to the decrease in side-chain size from a valine to an alanine in V44A. The error bars are standard deviations that are derived from a Monte Carlo simulation assuming Gaussian distribution of random error in peak heights. (b) Novel mechanism of how FAD mutation V44M and V44A increase Aβ42/Aβ40 ratio. V44M and V44A open up T48 for the initial ε-cleavage by γ-secretase. The change in Aβ product line preference towards Aβ42 by FAD mutations increases Aβ42/Aβ40 ratio. Figure 5: HD exchange shows that FAD mutants V44M and V44A destabilize the local conformations of T48 more than L49. ( a ) HD exchange rates for slowly exchanging residues in WT APPTM, V44M and V44A are plotted. Terminal residues (K28-M35 and L52-K55) exchange with D 2 O completely within 1 h ( k ex >5 per h) and their rates are not plotted. Exchange rates for T48 are significantly enhanced by V44A and V44M mutations while the increases for L49 are to a lesser extent. Increased k ex values at A44 and T43 are likely due to the decrease in side-chain size from a valine to an alanine in V44A. The error bars are standard deviations that are derived from a Monte Carlo simulation assuming Gaussian distribution of random error in peak heights. ( b ) Novel mechanism of how FAD mutation V44M and V44A increase Aβ42/Aβ40 ratio. V44M and V44A open up T48 for the initial ε-cleavage by γ-secretase. The change in Aβ product line preference towards Aβ42 by FAD mutations increases Aβ42/Aβ40 ratio. Full size image HD exchange experiment was also carried out for V44A, another FAD mutant. In V44A, T48 has a 4 fold enhancement in k ex , increasing from 0.009 per h in WT to 0.036 per h in V44A ( Fig. 5a ), while L49 has only an ~30% fold increase (0.028 per h in WT versus 0.036 per h in V44M) ( Fig. 5a ). Such changes in k ex may indicate enhanced accessibility of T48 site to ε-cleavage by γ-secretase. Indeed, it has been reported recently that V44A dramatically increase the ratio of AICD49-99/AICD50-99 (ref. 34 ), where AICD49-99 and AICD50-99 are the product of ε-cleavage at L48 and T49, respectively. For the first time, we have compared the structure and dynamics of WT APPTM and one of its FAD mutants V44M at atomic resolution. We find that V44M mutation destabilizes the local helical conformation and increases dynamics at the ε-cleavage sites. These changes are especially pronounced for T48, the initial ε-cleavage site for the Aβ42 production, as shown by the large amide proton CSP, lengthening of the helical hydrogen bonds and significantly amplified k ex . Similar changes in CSP and HD exchange rate were obtained for V44A, another FAD mutant. These data indicate that T48 is much more prone to undergo helical unwinding in V44M and V44A than WT, suggesting a structural mechanism of how V44M and V44A can increase Aβ42/Aβ40 ratio ( Fig. 5b ). γ-Secretase first cleaves APPTM endoproteolytically at the ε-sites, at residues T48 or L49 (refs 14 , 35 , 36 ), followed by carboxypeptidase-like activity, resulting in two lines of Aβ production: the Aβ42 line (48→45→42→38), and Aβ40 line (49→46→43→40) ( Supplementary Fig. S1 ). For the initial ε-cleavage to occur, the ε-site scissile bonds need to be accessible to the γ-secretase active site and catalytic water, which requires the unraveling of the local helical conformation. Because the T48 and L49 amides are adjacent to the scissile bond carbonyl within the same residue, these amides serve as excellent reporter for the accessibility of the ε-sites. While the V44M and V44A mutations destabilize the local helical conformation of both ε-cleavage sites, the mutations destabilizes the T48 site more than L49 site. The increased accessibility of T48 for ε-cleavage can shift Aβ production towards Aβ42, increasing the Aβ42/Aβ40 ratio. Such increased accessibility of T48 for ε-cleavage will lead to enhanced ε-cleavage at T48 relative to T49. This has been recently demonstrated by Dimitrov et al ., who reported a dramatic enhancement in the ratio of AICD49-99/AICD50-99 in V44A and other FAD mutants near the γ-secretase cleavage site [34] . The proposed mechanistic hypothesis is also consistent with the report that FAD mutations within APP usually increase the Aβ42/Aβ40 ratio by modifying the product line preference of γ-secretase [35] . An alternate dimer structure of APPTM WT was reported in early 2012 by Nadezhdin et al . [28] This structure was also solved in DPC micelles and exhibited a similar dimer interface as in our structure, with the GXXXA as the dimerization motif. The Nadezhdin structure is significantly different from our structure, as the RDC values used in our structure calculation are not consistent with the Nadezhdin structure ( Supplementary Fig. S7 ). A major difference between our structure and the Nadezhdin structure is that we have a right-handed dimer, while they have a left-handed dimer. Their construct contained an additional 13 residues QKLVFFAEDDVGS to the N-terminus of APPTM, which formed a nascent helix and could contribute to the structural discrepancy. Their dimer structures were built on 6 intermolecular NOEs between methyl groups from filtered experiments only. In contrast, our structures are based upon intermolecular NOEs derived from three differentially labelled NMR chimera samples, in addition to NOEs from filtered experiments ( Fig. 2 ). We used a mixed sample of [U- 15 N; U- 2 H] APPTM and unlabelled APPTM to obtain intermolecular NH-methyl NOEs. We also utilized a 1:1 mixture of [U- 15 N] labelled and [U- 13 C] labelled sample to yield unambiguous intermolecular NOEs between 15 N-H and 13 C-H. No RDC data were used in the calculation of the Nadezhdin structure while our structures were refined with RDCs determined in two alignment media, dGpG and stretched gel. RDC values can globally define NH orientations and avoid potential mistakes resulting from the local nature of NOE distance constraints. A recent NMR structure of C99 has been published which includes APPTM within the sequence [23] . C99 is known to dimerize through APPTM and is present in both monomer and dimer forms [24] , [31] , [37] . Barrett et al . chose to solve the monomer structure of C99 in lyso-myristoylphosphatidylglycerol (LMPG) micelles and primarily focused on the cholesterol-binding properties of C99. Therefore, the C99 NMR structure represents an alternative functional state for APPTM from our APPTM dimer structure. Interestingly, Barrett et al . showed that one of the GXXXG motifs plays a key role in cholesterol binding, which is consistent with our observation that GXXXG motif is not involved in APPTM dimerization. APPTM dimerization has been well-established, but the dimerization motif has been controversial. There are three potential dimerization motifs within APPTM: two GXXXG motifs and one GXXXA motif ( Supplementary Fig. S1 ). Several groups provided evidence supporting GXXXG motifs as the key dimerization motif [25] , [27] , [31] , [38] , [39] , while the current study, Nadezhdin et al . [28] and Gorman et al . [26] demonstrated that the GXXXA motif is the single most important motif for dimerization. The differences in the literature are likely due to variations in experimental conditions. Disparate membrane mimetics, for example, the different types of detergent, lipid and membrane system employed, can have dramatic impact on the dimerization mode. Indeed a solid-state NMR study has shown that lipid composition in multi-lamellar vesicle can significantly alter the conformation and dynamics of APPTM [29] . Recently, Wang et al . published an MD simulation of APPTM dimerization in conjunction with TOXCAT dimerization assay and showed that APPTM may have multiple dimerization modes, in which both GXXXG and GXXXA can mediate dimerization [31] . Therefore, it is likely that APPTM may dimerize through various motifs under different physiological conditions and for different functions. The presence of cholesterol may induce a dimerization mode more amenable to γ-secretase cleavage, where GXXXA mediates dimerization and GXXXG motifs bind to cholesterol. As the γ-secretase cleavage progresses and the hydrophobicity of APPTM decreases, the dimerization motif may shift towards the N-terminus and be mediated by the GXXXG motifs, facilitating the exit of Aβ from the membrane. In summary, we have shown that the V44M and V44A FAD mutations change the structure and dynamics of ε-cleavage sites. T48, the ε-cleavage site for Aβ42 generation, is likely more accessible to γ-secretase in the V44M and V44A mutants, leading to a shift towards the Aβ42 production line and to increased Aβ42/Aβ40 ratio. Such a structural mechanism may be applicable for other FAD mutants within APPTM and suggests that the ε-cleavage site may be a promising target for AD drug discovery. Materials Isotopically labelled compounds necessary for APPTM NMR sample production, such as 2 H-labelled DPC, were purchased from Cambridge Isotope Laboratories. Protein expression and purification The APPTM gene was cloned into the pETM41 vector for expression as an MBP fusion protein and purified by an amylose affinity column followed by TEV protease digest [32] . The FAD mutants, V44M and V44A of APPTM was obtained through site-directed mutagenesis. NMR spectroscopy The NMR sample contains 0.2–0.5 mM of APPTM with 5% DPC, 25 mM sodium phosphate at pH 7.2 and 10% D 2 O. NMR experiments for assignment and structure calculation were performed on either a 600 or 800 MHz Bruker Advance II spectrometer equipped with cryogenic probes, at 313 K. Spectra were processed with nmrPipe software [40] and analysed using Sparky (T.D. Goddard and D.G. Kneller, SPARKY 3, University of California, San Francisco, CA). For APPTM WT and V44M, the backbone resonances were assigned using HNCACB and HNCOCACB. Side-chain assignments were carried out using 15 N-TOCSY, (H)C(CCO)NH-TOCSY, H(CCCO)NH-TOCSY and HC(C)H-TOCSY experiments. Stereospecific assignment of side-chain valine and leucine was obtained by fractional 10% 13 C labelling. Assignments of ε-methyls of methionines were accomplished by mutagenesis. Backbone assignment of V44A was obtained by an HNCA experiment. NMR structure determination CYANA3.0 (ref. 41 ) was used for initial structure calculation. Distance constraints were obtained from 13 C and 15 N-NOESY spectra. Intermolecular NOEs were specifically detected by both filtered experiments and appropriate experiments for chimera NMR samples ( Fig. 2 ). The structure from CYANA with the lowest target function values were subject to refinement using XPLOR-NIH [42] with RDC from stretched gel [43] and d(GpG) [44] . The quality of the final structures was assessed with PSVS [45] . 20 lowest energy conformers out of 200 refined structures were deposited into protein data bank (2LZ3 and 2LZ4). Ramanchandran statistics for the 20 structures are 95.2% and 95.1% in the most favoured regions, 4.8% and 4.9% in the additionally allowed regions for WT and V44M, respectively, 0% in either generally allowed or disallowed regions. HD exchange APPTM were exchanged into D 2 O using Zeba Spin Desalting Columns (Thermo Scientific). Samples were then monitored by 15 N– 1 H HSQC for up to 30 h at pH 7.2 and 298 K. Accession codes: The NMR structural coordinates and constraints of the wild-type and V44M APP-TM proteins have been deposited in the protein databank under accession codes 2LZ3 (WT) and 2LZ4 (V44M). How to cite this article: Chen, W. et al . Familial Alzheimer’s mutations within APPTM increase Aβ42 production by enhancing accessibility of ε-cleavage site. Nat. Commun. 5:3037 doi: 10.1038/ncomms4037 (2014).